Deterministic quasi-random nanostructures for photon control Controlling the flux of photons is crucial in many areas of science and technology. Artificial materials with nano-scale modulation of the refractive index, such as photonic crystals, are able to exercise such control and have opened exciting new possibilities for light manipulation. An interesting alternative to such periodic structures is the class of materials known as quasi-crystals, which offer unique advantages such as richer Fourier spectra. Here we introduce a novel approach for designing such richer Fourier spectra, by using a periodic structure that allows us to control its Fourier components almost at will. Our approach is based on binary gratings, which makes the structures easy to replicate and to tailor towards specific applications. As an example, we show how these structures can be employed to achieve highly efficient broad-band light trapping in thin films that approach the theoretical (Lambertian) limit, a problem of crucial importance for photovoltaics. Photon manipulation is of paramount importance in many areas of science and technology, such as energy harvesting [1] , sensing and imaging in the life-sciences [2] and in optical communications [3] , [4] . Photonic crystals are periodic structures that have opened un-precedent possibilities for confining and manipulating light [4] , [5] , [6] , [7] . Such structures are essential building blocks in photonics that have given rise to key devices such as distributed feedback lasers, Bragg mirrors and grating spectrometers. Their diffractive properties are dependent on their Fourier spectra, which tend to consist of a series of sharp peaks indicating their strong resonances for specific angles and wavelengths. As an alternative to periodic structures, quasi-crystals offer unique advantages such as higher point group symmetry [5] , [8] , [9] , [10] and richer Fourier spectra [9] , [10] , [11] . If broad-band operation is required, for example, for the out-coupling of light from light-emitting diodes (LEDs) [12] and for broad-band, broad-angle light trapping in solar cells, quasi-crystalline and random structures offer advantages due to their richer Fourier spectra [13] , [14] . Examples of quasi-crystalline structures include classical architectures such as the Fibonacci sequence [11] and the Penrose lattice [9] , while random structures include the range from randomised periodic [13] all the way to ‘amorphous’ [12] , [14] structures. The difficulty with quasi-crystalline and random structures is that their properties are difficult to tailor towards specific applications, as they are far less deterministic and lack the design tools available with periodic structures. In this article, we propose to solve this problem by exploring a class of structures that combines the rich spatial frequencies associated with quasi-crystals and random structures with the high level of control afforded by periodic structures. We term these structures ‘quasi-random’, as they appear random at first sight, yet they are periodic based on an extended unit cell ( Fig. 1 ); quasi-random materials have periodic lattices that exhibit spatial frequency properties characteristic of random structures. As an example, we investigate the use of a quasi-random structure for broad-band light trapping in thin film solar cells and we show that, by combining the advantages of both periodic and random domains, a quasi-random structure achieves broad-band light trapping efficiency that reaches 98% of the theoretical (Lambertian) limit [15] . 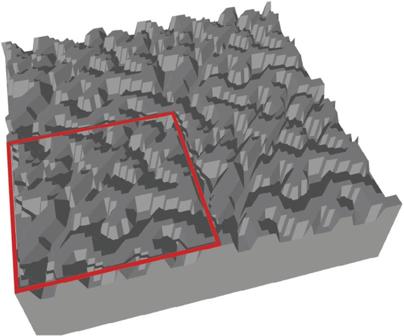Figure 1: Example of a quasi-random structure. The pattern is based on a modulated unit cell (highlighted) and a mesoscopic period of 1,800 nm. The mesoscopic period provides many Fourier components and the modulation controls the energy spread of these components. In this way, the rich Fourier spectra associated with quasi-crystals and random structures can be controlled in a deterministic way to suit different applications. Figure 1: Example of a quasi-random structure. The pattern is based on a modulated unit cell (highlighted) and a mesoscopic period of 1,800 nm. The mesoscopic period provides many Fourier components and the modulation controls the energy spread of these components. In this way, the rich Fourier spectra associated with quasi-crystals and random structures can be controlled in a deterministic way to suit different applications. Full size image Quasi-random designs Quasi-random structures are periodic, but with a period long enough to provide many Fourier components, thus giving the ‘appearance’ of a continuous spectrum. This property is achieved with mesoscopic periods, that is, periods typically 2–10 times greater than the operating wavelength. Their spatial frequency distribution is controlled via a deterministic and well-defined modulation of the unit cell that results in a supercell geometry. Interestingly, quasi-random structures follow the recent trend of exploring light propagation in diffusive materials; while adaptive optics principles may be used to recover the image information lost in a random medium [16] , we use the inverse process of controlling diffusion for increasing the viewing angle of a display device or a solar cell. Hence, understanding and controlling optical randomness is scientifically curious and technologically important. 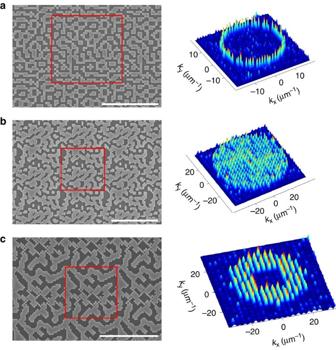Figure 2: Examples of quasi-random cells. Each cell was designed to concentrate the spectral energy into different regions in k-space. The scale bars of (a), (b) and (c) are 4 μm, 2 μm and 2 μm, respectively. (a) Periodic lattice with ring-shaped Fourier spectrum. This kind of structure is found in some biological systems and has also been used to extract light from organic light emitting diodes. (b) Lattice with Fourier energy concentrated into a well-defined circular region. This structure could be used in broad-band out-couplers, quasi-Lambertian scatterers or to provide broad-band feedback in distributed feedback lasers. (c) Quasi-random cell designed to suppress low orders and concentrate the energy into orders that can excite quasi-guided modes. This design is useful for light-trapping applications, as shown inFigs 3,4. Figure 2 shows some examples of modulated unit cells designed to control diffraction. These examples highlight the many opportunities offered by modulating a periodic single-level binary pattern that is directly amenable to mass-manufacturing, for example, by nanoimprint lithography. Figure 2: Examples of quasi-random cells. Each cell was designed to concentrate the spectral energy into different regions in k-space. The scale bars of ( a ), ( b ) and ( c ) are 4 μm, 2 μm and 2 μm, respectively. ( a ) Periodic lattice with ring-shaped Fourier spectrum. This kind of structure is found in some biological systems and has also been used to extract light from organic light emitting diodes. ( b ) Lattice with Fourier energy concentrated into a well-defined circular region. This structure could be used in broad-band out-couplers, quasi-Lambertian scatterers or to provide broad-band feedback in distributed feedback lasers. ( c ) Quasi-random cell designed to suppress low orders and concentrate the energy into orders that can excite quasi-guided modes. This design is useful for light-trapping applications, as shown in Figs 3 , 4 . Full size image The potential range of applications of such quasi-random structures is many-fold. For example, the colours of many biological systems are determined by complex epidermal photonic nano-structures [17] that are very challenging to replicate artificially [17] . The quasi-random structures we propose offer a unique opportunity for replicating such spectra. For example, the dragon fly [18] has an amorphous photonic structure with a well-defined ring-shaped Fourier energy distribution. A spectrum with such characteristics can be deterministically obtained with the quasi-random cell, as shown in Fig. 2a . The deterministic aspect of our quasi-random approach offers full control over the spectrum, for example, the radius of the ring. Such ring-shaped Fourier spectrum can also be employed as light output couplers in LEDs [12] . As a second example, the quasi-random structure of Fig. 2b exhibits a Fourier spectrum confined to a circular range of k-vectors. The region of energy concentration can be chosen to optimize light extraction from broad-band LEDs such as white organic LEDs [19] , or could be employed to create pseudo-random lasers [11] . Quasi-random structures for light trapping Third, a quasi-random structure can be used for the important problem of light trapping in thin film solar cells. In order to enhance light absorption, this type of solar cell employs nanostructures to couple light into the quasi-guided modes of its thin absorbing film [1] , [13] , [14] , [20] , [21] , [22] , [23] , [24] , [25] , [26] , [27] , [28] , [29] , [30] , [31] , [32] , [33] , [34] . The quasi-guided modes are usually excited by wavelength-scale periodic structures such as nano-wires [30] , [31] , photonic crystals [20] , [21] , [22] , [23] , [24] , [25] , [26] , [27] , [28] , [29] or metallic gratings [32] , [34] . The excitation of a quasi-guided mode results in strong resonant absorption enhancement, but only over a narrow bandwidth. A random structure, in contrast, offers broad-band, but weak enhancement [13] . The quasi-random cell of Fig. 2c offers a ‘sweet-spot’ in-between periodic and random domains by taking advantage of both; more resonances can be excited by its mesoscopic unit cell than by a wavelength-scale unit cell, yet these resonances are still strong because the modulation is designed to channel the diffracted energy only into the diffraction orders that can excite quasi-guided modes [29] . The boundary in k-space between components that can and cannot excite quasi-guided modes is defined by the light line. As the light line is wavelength-dependent, a wavelength has to be selected in order to define the radius of low k-values in Fourier space ( Fig. 2c ). Here we chose the operating wavelength to be λ 0 =600 nm because this is the point where absorption in silicon becomes critically weak. The corresponding k-vector component defined by the light line at 600 nm is |k| =10.5 μm −1 . Thus, we designed the quasi-random cell of Fig. 2c to have low diffraction efficiency for |k| <10.5 μm −1 . We then empirically chose a period of three times λ 0 , that is, a =1,800 nm for the quasi-random unit cell. 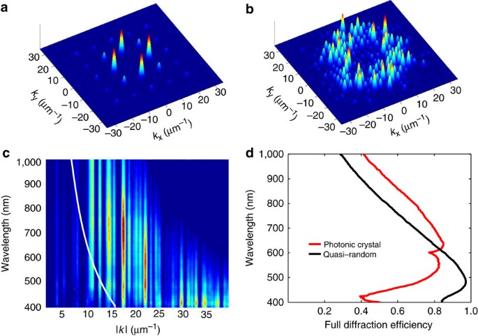Figure 3: Diffraction efficiency into silicon. The diffraction efficiency was calculated with the RCWA. (a) Diffraction efficiency of a 600 nm period photonic crystal. (b) Diffraction efficiency of the 1,800 nm period quasi-random structure ofFig. 2c. (c) Diffraction efficiency of the quasi-random structure ofFig. 2cas a function of k-vector amplitude (xaxis) and wavelength (yaxis). (d) FDE is defined as the total amount of energy in all orders other than the 0 order. The FDE is not greatly affected by the type of pattern used. The spectra of (a,b) were calculated for an excitation wavelength of 600 nm and a groove depth of 100 nm. The white line represents the light line. Figure 3 shows the diffraction efficiencies into silicon for (a) a photonic crystal with a period of 600 nm and (b) the quasi-random cell of Fig. 2c with a period of 1,800 nm. The depth of the grooves is 100 nm for both structures, which is a typical depth used in silicon–air interfaces for light trapping [29] . The spectra were calculated with the rigorous coupled wave analysis (RCWA) [35] . The benefit of using the quasi-random cell becomes clear by comparing Fig. 3a,b . The photonic crystal ( Fig. 3a ) diffracts light into only a few orders, which limits the excitation of quasi-guided modes. The quasi-random structure ( Fig. 3b ), in contrast, diffracts light into many orders and concentrates the diffraction energy only into those orders that can excite quasi-guided modes. In the limit of weak modulation (small refractive index contrast), the diffraction efficiency in Fig. 3b coincides with the Fourier transform shown in Fig. 2c . A comparison between the Fourier transform ( Fig. 2c ) and the diffraction efficiency ( Fig. 3b ) shows that the desired effect of concentrating the light into the higher orders is clearly maintained even for the strong refractive index contrast between silicon and air. Importantly, this effect is extended across a broad spectral range, as can be seen in Fig. 3c , which shows the diffraction efficiency as a function of wavelength and magnitude of k-vector |k| . Note that the light line, shown as the white line in Fig. 3c , delineates the boundary between low and high diffraction efficiency at the wavelength of 600 nm, which is the operating wavelength used in the design. The full diffraction efficiency (FDE), which is defined as the total amount of energy in all diffraction orders other than the 0 order, is shown in Fig. 3d . The FDE of the photonic crystal and the quasi-random surfaces are very similar: both reach a maximum in the short-wavelength region and slowly decay towards the infra-red. The FDE depends mostly on the refractive index contrast, groove depth and filling factor of the scattering medium and is therefore not greatly affected by the specific geometry used. The key point about the quasi-random cell is that it channels the diffracted energy into the desired modes. Figure 3: Diffraction efficiency into silicon. The diffraction efficiency was calculated with the RCWA. ( a ) Diffraction efficiency of a 600 nm period photonic crystal. ( b ) Diffraction efficiency of the 1,800 nm period quasi-random structure of Fig. 2c . ( c ) Diffraction efficiency of the quasi-random structure of Fig. 2c as a function of k-vector amplitude ( x axis) and wavelength ( y axis). ( d ) FDE is defined as the total amount of energy in all orders other than the 0 order. The FDE is not greatly affected by the type of pattern used. The spectra of ( a , b ) were calculated for an excitation wavelength of 600 nm and a groove depth of 100 nm. The white line represents the light line. Full size image The diffraction properties of the quasi-random cell provide a powerful light-trapping scheme. 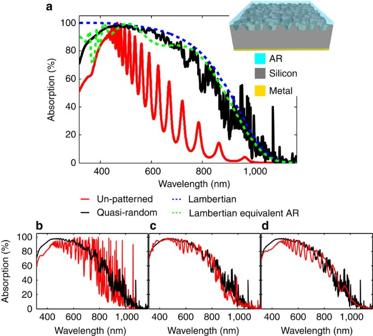Figure 4: Absorption spectra of nanostructured silicon thin films. (a) Absorption spectra of a 1 μm silicon thin film patterned by a quasi-random supercell (in black) and un-patterned (in red). The thin film is coated with a 70 nm AR coating and has a perfect conductor as the back electrode. The broad-band thin film absorption approaches the Lambertian limit across the entire spectrum of interest. (b) Comparison between a quasi-random structure (in black) and an optimized photonic crystal (in red). (c) Comparison between a quasi-random structure (in black) and a perturbed photonic crystal (in red). (d) Comparison between a quasi-random structure (in black) and an amorphous structure (in red). All spectra were calculated assuming un-polarized light. Figure 4a shows the calculated absorption of a 1 μm thick crystalline silicon layer coated by a 70 nm anti-reflection (AR) coating of refractive index of 1.65, as in a previous study [27] . The quasi-random cell ridges are made of silicon and its grooves are made of an AR material of index 1.65, as shown in the inset of Fig. 4 . Further, a perfect conductor is placed on the back of the cell as a contact. Figure 4: Absorption spectra of nanostructured silicon thin films. ( a ) Absorption spectra of a 1 μm silicon thin film patterned by a quasi-random supercell (in black) and un-patterned (in red). The thin film is coated with a 70 nm AR coating and has a perfect conductor as the back electrode. The broad-band thin film absorption approaches the Lambertian limit across the entire spectrum of interest. ( b ) Comparison between a quasi-random structure (in black) and an optimized photonic crystal (in red). ( c ) Comparison between a quasi-random structure (in black) and a perturbed photonic crystal (in red). ( d ) Comparison between a quasi-random structure (in black) and an amorphous structure (in red). All spectra were calculated assuming un-polarized light. Full size image The absorption spectrum is shown in Fig. 4a together with the corresponding Lambertian limits [15] and the spectrum of an un-patterned slab of the same thickness. The Lambertian limit is calculated for two cases: the dashed blue curve assumes 100% light transmission at the silicon–air interface (perfect AR coating, typically assumed in the theoretical derivation of the Lambertian limit), while the dashed green curve is calculated for the real transmission into the silicon layer [15] , which provides a more realistic reference. This ‘real transmission’ is calculated for a simulated AR coating, that is, a single layer of refractive index 1.65 and thickness 70 nm, which can also be identified by the thin film interference effects seen around 400 nm in the dashed green curve of Fig. 4a . The broad-band enhancement of the quasi-random structure allows the absorption spectrum to approach both Lambertian limits and even to exceed the Lambertian limit for real transmission in several narrow wavelength ranges. Indeed, as shown in Table 1 , the integrated absorption calculated using the tabulated AM1.5G spectrum is 98% of the real transmission Lambertian limit. This means that our quasi-random cell approaches the maximum possible absorption in the ray optics limit very closely. The dips in the absorption at 740, 800 and 900 nm are due to thin film interference that could be avoided with further design refinements, thus allowing us to approach the Lambertian limit even more closely. Importantly, such strong absorption is very tolerant against variations of the angle of incidence (see Supplementary Fig. S1 ). In order to better appreciate the origin of such high performance, the absorption spectrum of the quasi-random structure is plotted together with the absorption spectra of an optimized photonic crystal ( Fig. 4b ), a perturbed photonic crystal [13] ( Fig. 4c ) and an amorphous structure ( Fig. 4d ) [36] . The photonic crystal was optimized by performing a parameter search (see Methods section). As the plots highlight, the quasi-random structure provides the best performance across the entire spectral region, which is a consequence of its optimum Fourier spectrum (see also Supplementary Fig. S2 , Supplementary Fig. S3 and Supplementary Note 1 ). A summary of the results is shown in Table 1 (for results in different spectral regions, see Supplementary Tables S1–S3 ). In order to obtain an objective comparison, these results were obtained for the same material, material thickness and wavelength range. We note that very high absorption has also been achieved with three-dimensional (3D) structures [23] , [24] , [30] and nano-wires [28] . Such designs have excellent AR properties that could be combined with the quasi-random approach to further boost the absorption beyond the Lambertian limit. Table 1 Summary of light trapping performance. Full size table Experimental demonstration of a quasi-random design Finally, we test the practicality of the quasi-random structures by fabricating the cell of Fig. 2c into a 1 μm thick monocrystalline silicon thin film transferred to a glass substrate [37] . As the quasi-random cell is a diffracting element, an integrating sphere is used to collect the reflected, transmitted and diffracted light. Thus, the absorption can be calculated as , where n stands for the diffraction order, R for reflection and T for transmission. As shown in Fig. 5 , the match between theory and experiment is nearly perfect, thus validating the quasi-random approach and highlighting the applicability of the quasi-random cell for realistic devices. For comparison, we also calculate the Lambertian limit for the situation where no back-reflector is present, as is the case in this experiment. Encouragingly, the measured absorption also approaches the Lambertian limit for 100% transmission. 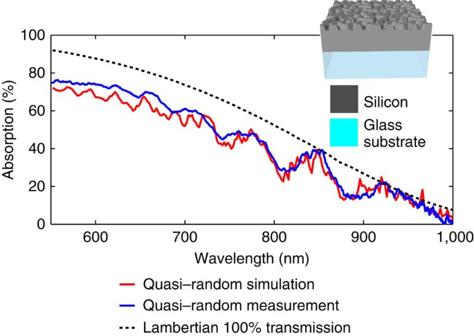Figure 5: Comparison between measured and calculated absorption spectra. The structure consists of a 1 μm silicon thin film sitting on a glass substrate and patterned with the quasi-random supercell. The grooves depth of the patterned layer is 110 nm and the pattern area is 1 × 1 mm2. Figure 5: Comparison between measured and calculated absorption spectra. The structure consists of a 1 μm silicon thin film sitting on a glass substrate and patterned with the quasi-random supercell. The grooves depth of the patterned layer is 110 nm and the pattern area is 1 × 1 mm 2 . Full size image We have introduced a class of materials we refer to as ‘quasi-random’ and explored their use for photon control. The structures are based on single-level binary gratings that are easy to design and to fabricate, yet they take advantage of the rich spectra of quasi-crystals and random structures that can be fully controlled. In this way, an extra degree of freedom is obtained to improve photon control. As an application example, the spectral characteristic of a quasi-random cell is designed to concentrate the diffracted energy into higher orders, which has important benefits for light trapping in solar cells. Owing to the combination of a mesoscopic period of 2–10 wavelengths and an optimized spectral distribution, the performance of this quasi-random cell was shown to approach the theoretical maximum (Lambertian limit) both theoretically and experimentally. Hence, we offer a simple solution for improving the efficiency of thin film solar cells without having to resort to multi-level or blazed gratings that are more difficult to make. The quasi-random cells could be employed in any application that benefits from the rich spectra of quasi-crystals such as artificial deterministic structures to replicate the scattering mechanisms of naturally occurring photonic structures or as broad-band light out-couplers for LEDs. Quasi-random structure designs The quasi-random structures were designed with a direct binary search in which the ridges and grooves are represented by a matrix of 0’s and 1’s. The binary search uses a target that expresses both the amount of energy into the desired Fourier orders and their uniformity. For example, the target functions used for the optimization shown in Fig. 2c are and , where A n is the amplitude of the Fourier coefficient n and n runs over the desired Fourier orders whereas m runs over all Fourier orders. The target was defined as T=(1−S 1 )B+S 2 , where B is a variable to define the balance between the targets (set to 0.5 for the quasi-random designs). A search is then performed by swapping the matrix elements and checking the target value. If the target decreased after swapping a given matrix element, the new element is held; otherwise, the change is discarded and the previous element is maintained. This method, even though it has already led to a structure that performs close to the Lambertian limit, may be improved further, especially if a more complex algorithm that assesses both local and global maxima is used. Diffraction efficiency and absorption calculation The diffraction efficiencies were calculated with the scattering matrix analysis, which is a version of the RCWA. The method was implemented as described in a previous study [35] . The method’s convergence depends on the period of the structure. The quasi-random (period of 1,800 nm) and the photonic crystal (period of 600 nm) required less than 441 and 121 plane waves to reach convergence, respectively. The absorption spectra of the photonic crystal and quasi-random structures were calculated with both RCWA and finite-difference time-domain (FDTD), and were verified against each other. The absorption spectra of the perturbed and amorphous structures were calculated with FDTD. Photonic crystal optimization The light-trapping properties of a photonic crystal combined with an AR coating of refractive index of 1.65 have previously been extensively investigated in ref. 27 . The optimization was carried out searching the maximum absorption by varying the hole radius, period and groove depth. The optimum condition for a 1 μm thick crystalline silicon slab is a period of 600 nm, a hole radius of 198 nm and a groove depth of 190 nm. These were the parameters used in the comparison with the quasi-random cell. Perturbed crystal and amorphous design The perturbed photonic crystal design was implemented following the optimized perturbation strength previously described [13] , which is 20% of the lattice constant. The amorphous structure design was taken from a previous study [36] and scaled so that the high energy ring coincides with the useful region for light trapping (see Supplementary Fig. S2 ). A 14 × 14 μm 2 unit cell was employed to simulate the amorphous structure. Silicon thin film fabrication Thin films of crystalline silicon of 1 μm thickness on glass were prepared by the epi-free method previously described [37] . The method creates a suspended film by annealing a silicon wafer (B-doped 20 Ωcm Cz) at 1,130 °C that has been patterned with regularly spaced cylindrical pores that were defined by deep-UV lithography and dry etching. The high temperature enables surface diffusion, and thus pore closure and merging into a single buried void, with a thin film above. The thickness of the film is controlled by the pore dimensions. The film is then transferred onto borosilicate glass by anodic bonding (300 °C, 1,000 V) of its top surface and detaches by itself from its parent silicon wafer. This bonding method results in a strong bond with a thin interfacial oxide of a few nanometres as a bonding agent. Silicon thin film patterning The thin films were patterned by electron beam lithography (ebeam) by the following procedure. First, an ebeam resist (ZEON ZEP 520A) was spin-coated onto the thin film. Second, the ebeam resist was patterned using a Leo/Raith Plus ebeam system and the resist was developed in xylene at 23 °C. The pattern was finally transferred into the silicon thin film by reactive ion etching using a mixture of CHF 3 and SF 6 (1:1). Absorption measurement The patterned thin film absorption was measured using an integrating sphere and a white light source (Koheras SuperK COMPACT) at an angle of incidence of 3° to ensure that the specularly reflected light does not escape through the entrance port. The spectrum was measured using an Ocean Optics Spectrometer (USB 2000) with wavelength resolution of <2 nm. How to cite this article: Martins, E. R. et al. Deterministic quasi-random nanostructures for photon control. Nat. Commun. 4:2665 doi: 10.1038/ncomms3665 (2013).